Cadmium iodide-mediated allenylation of terminal alkynes with ketones Allenes are important building blocks in organic synthesis and have attracted much attention from researchers worldwide. So far, mono- and 1,3-disubstituted allenes can be prepared easily by applying the allenylation of terminal alkynes reaction of aldehydes. However, trisubstituted allenes have never been reported using this reaction due to the extremely low reactivity of ketones. Here, we report the one-pot synthesis of trisubstituted allenes from terminal alkynes and ketones utilizing cadmium iodide as the mediator. With this protocol, a series of different allenes, including 1,5-bisallenes and optically active allenols, which are especially important in synthetic chemistry, have been successfully prepared. Allene moieties have been found in many natural products and pharmaceuticals [1] , [2] , [3] , [4] . Due to the unique reactivities, allenes have also been demonstrated as useful and important starting materials in organic synthesis [5] , [6] , [7] , [8] , [9] , [10] , [11] , [12] , [13] , [14] , [15] , [16] , [17] , [18] , [19] , [20] , [21] , [22] , [23] , [24] , [25] . Thus, efficient methods for the synthesis of allenes from simple and readily available chemicals are highly desirable [26] , [27] , [28] , [29] , [30] , [31] , [32] , [33] , [34] , [35] , [36] . For such a reaction, the most straight forward method is using the allenylation of terminal alkynes (ATA) reaction due to the fact that all the starting materials, that is, terminal alkynes, amines, carbonyl compounds (aldehydes and ketones), are common chemicals in any chemical laboratory [37] , [38] , [39] , [40] , [41] . However, so far this ATA reaction may only be applied to paraformaldehyde (with Cu I ) [37] , [38] , [39] , [40] and aldehydes (with Zn II or Cu(I)) [41] for the synthesis of mono- and 1,3-disubstituted allenes. The synthesis of trisubstituted allenes from this approach using ketones is still not possible ( Fig. 1 ) [42] , [43] . 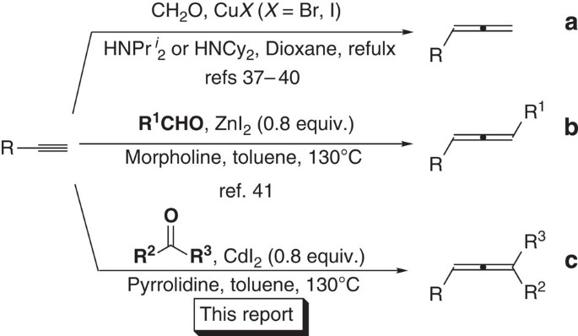Figure 1: Approaches to allenes from terminal alkynes. (a) Allenylation using formaldehdye. (b) Allenylation using aldehydes. (c) Synthesis of trisubstituted allenes using ketones. Figure 1: Approaches to allenes from terminal alkynes. ( a ) Allenylation using formaldehdye. ( b ) Allenylation using aldehydes. ( c ) Synthesis of trisubstituted allenes using ketones. Full size image In this paper, we report a method for the synthesis of trisubstituted allenes using a CdI 2 (refs 44 , 45 )-mediated ATA reaction of ketones ( Fig. 1 ). With the use of CdI 2 , a series of trisubstituted allenes can be prepared easily in a one-pot synthesis. By applying this protocol, 1,5-bisallenes and optically active allenols, which are useful in organic synthesis, can also be prepared successfully. Different inorganic metallic salts for the ATA reaction Our initial work began with commercially available starting materials: phenylacetylene 1a , 2-hexanone 2a and pyrrolidine 3a under the mediation of different groups 11 and 12 inorganic metallic salts ( Table 1 ). After systematic trials, we were happy to find that the ATA reaction of 1a (1.0 mmol) and 2a (1.1 mmol) in the presence of pyrrolidine 3a (1.1 mmol) with CdI 2 (0.8 mmol) in 5 ml of toluene with stirring at 130 °C for 4 h afforded the trisubstituted allene 4a in 57% yield ( Table 1 , entry 4)! Other metallic salts in groups 11 and 12, such as CuI (refs 37 , 38 , 39 , 40 , 46) , ZnI 2 (ref. 41 ), AgI (ref. 47 ), AuI (ref. 48 ) and HgCl 2 , afforded only a trace amount of the expected trisubstituted allene 4a ( Table 1 , entries 1–3, 5 and 6). Table 1 Group 11 or 12 metal salts for ATA reaction * . 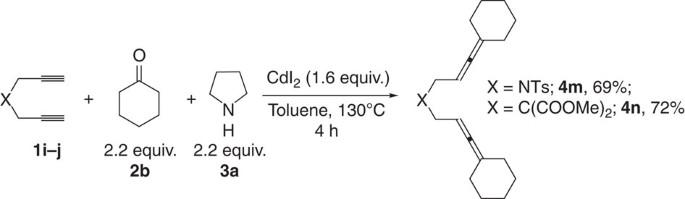Figure 2: Synthesis of 1,5-bisallenes with ATA reaction. 1,5-Bisallenes were synthesized by applying this protocol, which are not easily prepared by other methods. NTs=N-tosyl. Full size table Optimization of the ATA reaction The reaction was sensitive to the concentration of the substrates ( Table 2 , entries 1–3). With 0.6 equiv. of CdI 2 , the yield dropped dramatically ( Table 2 , entry 4). We also examined the solvent effect, with toluene still being the best ( Table 2 , entry 5). The yield of trisubstituted allene 4a with CdBr 2 was only 7% ( Table 2 , entry 6). Thus, 1a (1.0 mmol), 2a (1.1 mmol), 3a (1.1 mmol) and CdI 2 (0.8 mmol) in 5 ml of toluene with stirring at 130 °C for 4 h were defined as the optimized reaction conditions for further study, as the same reaction at 120 °C gave a lower yield (46%). Table 2 Optimization of ATA reaction conditions * . 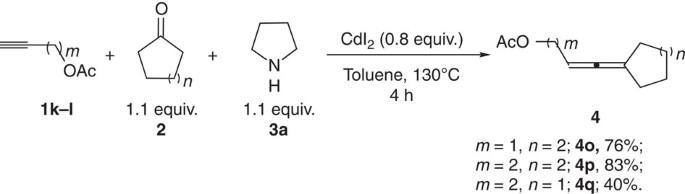Figure 3: Synthesis of acetyl-protected trisubstitutedα- andβ-allenols. Easily available acetyl-protected propargyl alcohols could be converted to trisubstituted allenes using ATA reaction. Full size table Substrate scope With the optimal reaction conditions in hand, we then investigated the scope of the reaction by applying various terminal alkynes and ketones ( Table 3 ). First, differently substituted terminal aryl-substituted alkynes were examined. Phenylacetylene 1a and the analogues substituted with p -MeO, p -Br, m -Br and o -Cl groups all afforded good yields of the products, providing further opportunity of elaboration ( Table 3 , entries 1–5). Heteroaryl-substituted acetylene 1f was also suitable for this reaction with 41% yield ( Table 3 , entry 6). The reaction may also be extended to terminal alkyl-substituted alkynes such as 1-octyne 1g and 1-decyne 1h , which gave trisubstituted allenes 4h and 4i in 82% and 80% yields, respectively ( Table 3 , entries 7 and 8). Next, we turned to investigate the ATA reaction with different ketones. 2-Hexanone 2a reacted with phenylacetylene 1a to give the corresponding allene 4a in 55% yield ( Table 3 , entry 9); 2-octanone 2c and 4-phenyl-2-butanone 2d worked well with 1-octyne 1g and 1-decyne 1h to afford the corresponding allenes 4k and 4l in 63% and 54% yields, respectively ( Table 3 , entries 11 and 12). Table 3 The scope of terminal alkynes and ketones * . Full size table Synthesis of 1,5-bisallenes As we know, 1,5-bisallenes are useful starting materials in organic synthesis [20] , [49] . With this methodology, 1,5-bisallenes 4m and 4n could be easily prepared in 69% and 72% yields ( Fig. 2 ). Figure 2: Synthesis of 1,5-bisallenes with ATA reaction. 1,5-Bisallenes were synthesized by applying this protocol, which are not easily prepared by other methods. NTs= N -tosyl. Full size image Synthesis of acetyl-protected α - and β -allenols Recently, allenols have been proven as versatile building blocks in organic synthesis [5] , [50] , [51] , [52] , [53] . By applying this protocol, acetate-protected trisubstituted α - and β -allenols could be obtained in moderate to good yields ( Fig. 3 ). Figure 3: Synthesis of acetyl-protected trisubstituted α - and β -allenols. Easily available acetyl-protected propargyl alcohols could be converted to trisubstituted allenes using ATA reaction. Full size image Preparation of trisubstituted allene on gram scale It is easy to conduct the reaction on a 1-g scale to afford 4r in 50% yield, which could be easily deprotected by its treatment with K 2 CO 3 in MeOH and H 2 O to afford the corresponding allenol 4s in 96% yield, indicating the potential synthetic utility of this method ( Fig. 4 ). 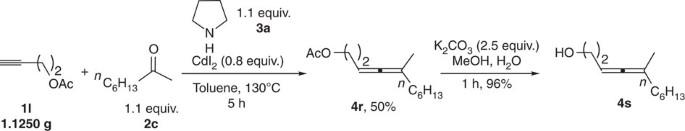Figure 4: Gram-scale synthesis of 5,5-disubstituted allenol4r. The reaction could be conducted on a 1-g scale to afford acetyl-protected trisubstituted allene, which could be converted to allenol easily. Figure 4: Gram-scale synthesis of 5,5-disubstituted allenol 4r . The reaction could be conducted on a 1-g scale to afford acetyl-protected trisubstituted allene, which could be converted to allenol easily. Full size image Trisubstituted allenes with central and/or axial chirality When we used the tert -butyldimethylsilyl ether of chiral alkynol ( S )- 1m (>99% ee) as the starting material, optically active tert -butyldimethylsilyl-protected α -allenol ( S )- 4t was also afforded in 87% yield with 99% ee ( Fig. 5a ). Nonsymmetrical ketone 2a was also suitable for this reaction yielded a pair of diastereoisomers (d.r.=1:1) in 69%, indicating that there is no 1,2-chiral induction of the propargylic central chirality on the in situ formed axial chirality ( Fig. 5b ). 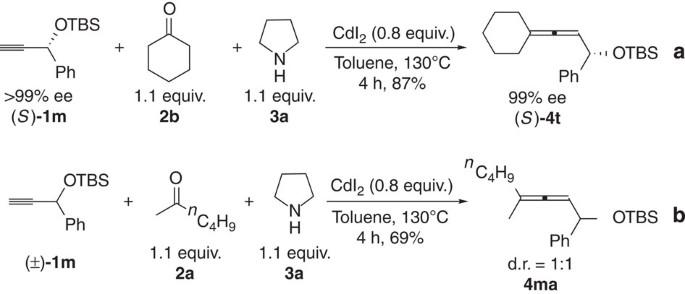Figure 5: ATA reaction with protected terminal propargylic alcohols. (a) When TBS-protected chiral alkynol was used, the chirality was kept in the allene product. (b) When nonsymmetrical keone2areacted with alkynol (±)−1 m, a pair of diastereoisomers were observed (d.r.=1:1). TBS,tert-butyldimethylsilyl. Figure 5: ATA reaction with protected terminal propargylic alcohols. ( a ) When TBS-protected chiral alkynol was used, the chirality was kept in the allene product. ( b ) When nonsymmetrical keone 2a reacted with alkynol (±)− 1 m , a pair of diastereoisomers were observed (d.r.=1:1). TBS, tert -butyldimethylsilyl. Full size image Intermediates It is observed that the reaction of phenylacetylene 1a , 2-octanone 2c and pyrrolidine 3a at a lower temperature, 100 °C, for 1 h afforded the corresponding propargylic amine 5j in 24% isolated yield with 3% 1 H NMR yield of allene 4j . Then propargylic amine 5j was converted to allene 4j in 82% yield under the standard reaction conditions, indicating the intermediacy of 5j- type propargylic amine in this type of reaction. What is more, the propargylic amines 5u–5x may be converted to the corresponding allenes 4u–4x in 45–88% yields in the presence of CdI 2 in toluene at 130 °C within 4 h ( Fig. 6 ). 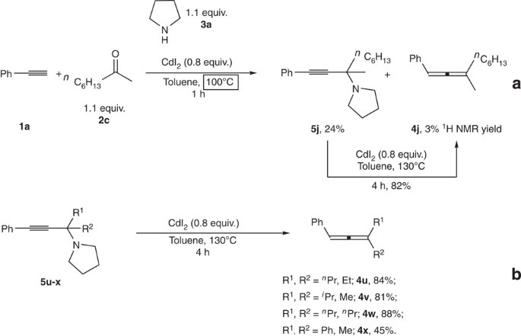Figure 6: Synthesis of allenes from propargylic amines. (a) The intermediate, propargylic amine5j, was synthesized at 100 °C and then converted to the allene successfully. (b) Allenylation of propargylic amines. Figure 6: Synthesis of allenes from propargylic amines. ( a ) The intermediate, propargylic amine 5j , was synthesized at 100 °C and then converted to the allene successfully. ( b ) Allenylation of propargylic amines. Full size image From the results in Table 1 , it should be noted that only in the case of CuI, propargylic amine 5a was formed in 73% yield, which could not be converted to allene 4a under the mediation of CuI ( Table 1 , entry 1), demonstrating that only CdI 2 is working for both the propargylic amine and allene formation steps. In fact, with this notion that CuI could mediate the formation of propargylic amine 5a , which was considered as the intermediate, a number of metallic salts, such as ZnI 2 , AgI, AuI and HgCl 2 , were tried in this reaction in the presence of CuI ( Table 4 ). Unfortunately, none of these mixed systems could mediate the formation of allene 4a in decent yield, indicating the unique effect of CdI 2 on this ATA reaction. Table 4 Mixed metal salts for ATA reaction * . Full size table Based on the above data and recent reports of this type of reactions [41] , [47] , we proposed a plausible mechanism for the ATA reaction ( Fig. 7 ): Alkynyl cadmium species 6 , generated from terminal alkyne in the presence of pyrrolidine, would react with the ketoniminum 7 formed in situ from ketone and pyrrolidine, to give the corresponding propargylic amine 5 . The carbon−carbon triple bond in propargylic amine 5 coordinates to CdI 2 forming complex 8 , which would be followed by 1,5-hydride transfer and β -elimination to afford the corresponding trisubstituted allene 4 . 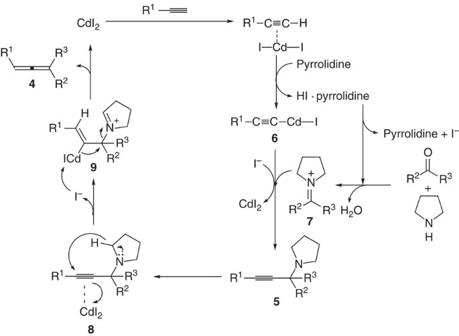Figure 7: Proposed mechanism for the ATA reaction of ketones. The key step of propargylic amine formation followed by 1,5-hydride transfer andβ-elimination. The intermediate, propargylic amine5j, was synthesized at a lower temperature and could be converted to the allene successfully. Figure 7: Proposed mechanism for the ATA reaction of ketones. The key step of propargylic amine formation followed by 1,5-hydride transfer and β -elimination. The intermediate, propargylic amine 5j , was synthesized at a lower temperature and could be converted to the allene successfully. Full size image In conclusion, we have developed an efficient CdI 2 -mediated ATA reaction to synthesize trisubstituted allenes from commercially available alkynes and ketones. This protocol is operationally simple and all the starting materials are basic chemicals readily available, showing the potential synthetic utility of this method. Further studies including the asymmetric version of this reaction and the application of these allenes are being conducted in our laboratory. Materials Chloroform- d (Cambridge Isotope Ltd.) for 1 H and 13 C NMR spectroscopy was used as received. CdI 2 (99.5%) was purchased from Aladdin and kept in a glove box. Toluene was dried over sodium wire with benzophenone as indicator and distilled freshly before use. Other reagents were used without further treatment. General spectroscopic methods 1 H NMR spectra were obtained at 27 °C using an Agilent spectrometer operating at 400 MHz. 13 C NMR spectra were obtained at 27 °C using an Aglient spectrometer operating at 100 MHz. 1 H NMR, 13 C NMR and HPLC spectra are supplied for all compounds: see Supplementary Figures S1–S56 . See Supplementary Methods for the characterization data of compounds not listed in this part. Synthesis of 1-phenyl-3-methyl-1,2-heptadiene 4a To a dried Schlenk tube was added CdI 2 (293.4 mg, 0.8 mmol) inside a glove box. The Schlenk tube was then taken out and dried under vacuum with a heating gun until the white CdI 2 turned to yellow green. 1a (101.5 mg, 1 mmol)/toluene (2.5 ml), 2a (109.8 mg, 1.1 mmol)/toluene (2.5 ml) and 3a (92.0 μl, d=0.852 g ml −1 , 78.3 mg, 1.1 mmol) were then added sequentially under Ar atmosphere. The Schlenk tube was then equipped with a condenser and placed in a pre-heated oil bath of 130 °C with stirring for 4 h. After cooling to room temperature, the crude reaction mixture was filtrated through a short pad of silica gel eluted with ether (20 ml). After evaporation, the residue was purified by chromatography on silica gel to afford 4a (ref. 54 ) (102.7 mg, 55%) (eluent: petroleum ether) as a liquid: thin-layer chromatography (TLC) (petroleum ether): R f =0.92; 1 H NMR (400 MHz, CDCl 3 ) δ 7.31−7.23 (m, 4H, Ar−H), 7.19−7.11 (m, 1H, Ar−H), 6.07−6.01 (m, 1H, CH=C), 2.12−2.02 (m, 2H, CH 2 ), 1.79 (d, J =2.8 Hz, 3H, CH 3 ), 1.52−1.29 (m, 4H, 2 × CH 2 ), 0.89 (t, J =7.2 Hz, 3H, CH 3 ); 13 C NMR (100 MHz, CDCl 3 ) δ 202.6, 136.1, 128.4, 126.5, 126.3, 103.7, 93.7, 33.8, 29.7, 22.4, 18.8, 13.9; MS (EI) m / z (%) 186 (M + , 1.61), 129 (100); IR (neat): ν =2957, 2927, 2858, 1951, 1598, 1496, 1462, 1259, 1071, 1025, cm −1 . Gram-scale synthesis of acetyl-protected β -allenol 4r To a dried three-necked bottle was added CdI 2 (2.9307, g, 8 mmol) inside a glove box. The three-necked bottle was then taken out and dried under vacuum with a heating gun until the white CdI 2 turned to yellow-green. 1l (1.1250, g, 10 mmol)/toluene (20 ml), 2c (1.4100, g, 11 mmol)/toluene (20 ml) and 3a (0.7839, g, 11 mmol)/toluene (10 ml) were then added sequentially under Ar atmosphere. The three-necked bottle was then equipped with a condenser and placed in a pre-heated oil bath of 130 °C with stirring. After 5 h, the reaction was complete as monitored by TLC, the resulting mixture was cooled to room temperature and filtrated through a short pad of silica gel eluted with ether (100 ml). After evaporation, the residue was purified by chromatography on silica gel to afford 4r (1.1283, g, 50%) (eluent: petroleum ether/ethyl ether=30/1) as a liquid: TLC (petroleum ether:ethyl acetate, 10:1 v/v): R f =0.80; 1 H NMR (400 MHz, CDCl 3 ) δ 5.03−4.94 (m, 1H, CH=C=C), 4.10 (t, J =6.8 Hz, 2H, OCH 2 ), 2.28 (q, J =6.7Hz, 2H, CH 2 ), 2.04 (s, 3H,CH 3 ), 1.91 (td, J =7.4 Hz, 2.5 Hz, 2H, CH 2 ), 1.66 (d, J =2.4 Hz, 3H, CH 3 ), 1.44−1.22 (m, 8H, 4 × CH 2 ), 0.88 (t, J =7.0 Hz, 3H, CH 3 ); 13 C NMR (100 MHz, CDCl 3 ) δ 201.9, 171.0, 100.3, 85.6, 63.8, 33.8, 31.7, 28.9, 28.6, 27.4, 22.6, 20.9, 19.1, 14.0; MS (EI) m / z (%) 224 (M + , 1.01), 94 (100); IR (neat): ν=2956, 2926, 2856, 1966, 1742, 1459, 1383, 1364, 1231, 1035, cm −1 ; HRMS ( m/z ): [M] + calcd. for C 14 H 24 O 2 , 224.1776; found, 224.1779. Synthesis of optically active allene ( S )- 4t from chiral alkyne Following the synthesis procedure of 4a : The reaction of CdI 2 (293.7 mg, 0.8 mmol), ( S ) -1m (246.6 mg, 1 mmol)/toluene (2.5 ml), 2b (108.6 mg, 1.1 mmol)/toluene (2.5 ml) and 3a (92.0 μl, d =0.852 g/ml, 78.3 mg, 1.1 mmol) afforded ( S ) -4t (285.1 mg, 87%) (eluent: petroleum ether) as a liquid: TLC (petroleum ether): R f =0.93; 99% ee (HPLC conditions: Chiralcel OJ−H column, CO 2 / i -PrOH=98/2, 1.5 ml/min, λ =214 nm, t R (major)=7.2 min, t R (minor)=6.9 min); [ α ] D 21.7 = +132.7 ( c =1.01, CHCl 3 ); 1 H NMR (400 MHz, CDCl 3 ) δ 7.36 (d, J= 7.6 Hz, 2H, Ar−H), 7.30 (t, J =7.6 Hz, 2H, Ar−H), 7.21 (t, J =7.2 Hz, 1H, Ar−H), 5.21 (d, J =7.2 Hz, 1H, OCH), 5.12-5.04 (m, 1H, CH=C=C), 2.16−2.07 (m, 4H, 2 × CH 2 ), 1.63−1.46 (m, 6H, 3 × CH 2 ), 0.93 (s, 9H, 3 × CH 3 ), 0.11 (s, 3H, CH 3 ), 0.07 (s, 3H, CH 3 ); 13 C NMR (100 MHz, CDCl 3 ) δ 197.6, 144.8, 127.9, 126.7, 125.7, 104.1, 94.7, 74.6, 31.4, 31.1, 27.3, 27.2, 26.0, 25.9, 18.3, −4.4, −4.9; MS (EI) m / z (%) 328 (M + , 1.01), 221 (100); IR (neat): ν =2928, 2887, 2855, 1966, 1492, 1469, 1447, 1252, 1084, 1062, 1006, cm −1 ; HRMS ( m/z ): [M] + calcd. for C 21 H 32 OSi, 328.2222; found, 328.2225. Synthesis of the intermediate 5j To a dried Schlenk tube was added CdI 2 (293.8 mg, 0.8 mmol) inside a glove box. The Schlenk tube was then taken out and dried under vacuum with a heating gun until the white CdI 2 turned to yellow green. 1a (102.6 mg, 1 mmol)/toluene (2.5 ml), 2c (141.3 mg, 1.1 mmol)/toluene (2.5 ml) and 3a (92.0 μl, d=0.852 g ml −1 , 78.3 mg, 1.1 mmol) were then added sequentially under Ar atmosphere. The Schlenk tube was then equipped with a condenser and placed in a pre-heated oil bath of 100 °C with stirring for 1 h. After cooling to room temperature, the crude reaction mixture was filtrated through a short pad of silica gel eluted with acetone (20 ml). After evaporation, to the residue was added 27.0 μl of CH 3 NO 2 as the internal standard for 1 H NMR analysis (29% 1 H NMR yield of 5j and 3% 1 H NMR yield of 4j ) and then purified by chromatography on silica gel to afford 5j (67.5 mg, 24%) (eluent:petroleum ether/ethyl acetate=200:2 ml to 200:4 ml, then 20:1, finally petroleum ether/ethyl acetate/Et 3 N=500 ml/50 ml/0.5 ml was applied to get the pure product) as a liquid:TLC (petroleum ether:ethyl acetate, 10:1 v/v): R f =0.20; 1 H NMR (400 MHz, CDCl 3 ) δ 7.45−7.38 (m, 2H, Ar−H), 7.33−7.23 (m, 3H, Ar−H), 2.85−2.73 (m, 4H, CH 2 NCH 2 ), 1.83−1.72 (m, 5H, 2 × CH 2 +one proton of CH 2 ), 1.71−1.61 (m, 1H, one proton of CH 2 ), 1.59−1.41 (m, 5H, CH 2 +CH 3 ), 1.37−1.28 (m, 6H, 3 × CH 2 ), 0.89 (t, J =6.4 Hz, 3H, CH 3 ); 13 C NMR (100 MHz, CDCl 3 ) δ 131.7, 128.1, 127.6, 123.6, 91.3, 84.3, 57.9, 47.7, 41.5, 31.8, 29.7, 25.8, 24.3, 23.6, 22.6, 14.1; MS (ESI) m / z 284 (M+H + ), 213 (M+H + -pyrrolidine); IR (neat): ν =2954, 2928, 2857, 2808, 1598, 1489, 1463, 1443, 1370, 1253, 1193, 1143, 1101, 1070, 1026, cm −1 ; HRMS ( m / z ):[M+H] + calcd. for C 20 H 30 N, 284.2373; found, 284.2373. Synthesis of allene 4j from propargylic amine To a dried Schlenk tube was added CdI 2 (293.5 mg, 0.8 mmol) inside a glove box. The Schlenk tube was then taken out and dried under vacuum with a heating gun until the white CdI 2 turned to yellow green. 5j (284.1 mg, 1 mmol) and toluene (5 ml) were then added under Ar atmosphere. The Schlenk tube was then equipped with a condenser and placed in a pre-heated oil bath of 130 °C with stirring for 4 h as monitored by TLC. After cooling to room temperature, the crude reaction mixture was filtrated through a short pad of silica gel eluted with ether (20 ml). After evaporation, the residue was purified by chromatography on silica gel to afford 4j (176.9 mg, 82%) (eluent: petroleum ether) as a liquid: TLC (petroleum ether): R f =0.94; 1 H NMR (400 MHz, CDCl 3 ) δ 7.32−7.25 (m, 4H, Ar−H), 7.20−7.12 (m, 1H, Ar−H), 6.07−6.01 (m, 1H, CH=C=C), 2.07 (td, J =7.4 Hz, 2.5 Hz, 2H, CH 2 ), 1.80 (d, J =2.8 Hz, 3H, CH 3 ), 1.52−1.44 (m, 2H, CH 2 ), 1.38−1.21 (m, 6H, 3 × CH 2 ), 0.86 (t, J =7.0 Hz, 3H, CH 3 ); 13 C NMR (100 MHz, CDCl 3 ) δ 202.7, 136.1, 128.4, 126.5, 126.3, 103.7, 93.8, 34.1, 31.7, 29.1, 27.5, 22.7, 18.8, 14.0. How to cite this article: Tang, X. et al . Cadmium iodide-mediated allenylation of alkynes with ketones. Nat. Commun. 4:2450 doi: 10.1038/ncomms3450 (2013).